miRNA-based buffering of the cobblestone–lissencephaly-associated extracellular matrix receptor dystroglycan via its alternative3′-UTR Many proteins are expressed dynamically during different stages of cellular life and the accuracy of protein amounts is critical for cell endurance. Therefore, cells should have a perceptive system that notifies about fluctuations in the amounts of certain components and an executive system that efficiently restores their precise levels. At least one mechanism that evolution has employed for this task is regulation of 3′-UTR length for microRNA targeting. Here we show that in Drosophila the microRNA complex miR-310s acts as an executive mechanism to buffer levels of the muscular dystrophy-associated extracellular matrix receptor dystroglycan via its alternative 3′-UTR . miR-310s gene expression fluctuates depending on dystroglycan amounts and nitric oxide signalling, which perceives dystroglycan levels and regulates microRNA gene expression. Aberrant levels of dystroglycan or deficiencies in miR-310s and nitric oxide signalling result in cobblestone brain appearance, resembling human lissencephaly type II phenotype. Developmental biologists typically are interested in phenotypes caused by gene loss-of-function; however, multiple stresses, unfavourable conditions, or developmental events can affect the precision of gene expression at the transcriptional level, resulting in altered protein levels. Elevated amounts of a critical protein can potentially be as deadly as its deficiency. In addition, the levels of numerous proteins constantly fluctuate due to different phases of cellular life, such as the cell cycle stage, cell shape rearrangements and motility. Many of the essential cellular functions are dependent on cell–extracellular matrix (ECM) contacts and are associated with cell shape reorganization [1] , [2] . The ECM provides signalling cues that coordinate multiple cell behaviour aspects to guarantee proper tissue formation and homeostasis [3] . The extracellular signals from the ECM to the cytoplasm are transmitted via ECM receptors (that is, integrins and dystroglycan) to activate specific signalling pathways inside the cell, modifying the gene expression programme. Conversely, changes inside the cell are transduced via these transmembrane proteins to adjust the surrounding ECM composition that in turn changes cell biochemistry [2] , [4] . The ECM constituents also establish a three-dimensional microenvironment that controls cell division and growth, survival and differentiation. As these processes are very dynamic, it suggests a need for a mechanism that restores proper levels of cell adhesion proteins. This mechanism should account for at least two major tasks: to sense abnormal levels of the protein and to send this information to induce a cellular response that will re-establish equilibrium. Dystroglycan (Dg) is a conserved critical ECM receptor that is responsible for processes relevant to total organism health. It is a key component of the dystrophin (Dys) glycoprotein complex (DGC), connecting the ECM to the actin cytoskeleton via the cytoplasmic protein Dys [5] , [6] , [7] . The DGC is best known for its association with a large group of inherited neuromuscular diseases, muscular dystrophies. Owing to the high occurrence of these sometimes fatal diseases, the majority of research has focused on the role of the DGC in providing mechanical stability to the muscle sarcolemma to resist the vigour of contraction [6] , [8] , [9] . However, the DGC not only offers strength to the muscle sarcolemma, but also it has crucial roles in central nervous system development, as many muscular dystrophy patients experience cognitive impairment and learning disability, and develop some behavioural and neuropsychiatric disorders [10] . In particular, abnormal interaction of Dg and the ECM results in the cobblestone brain, which is an odd malformation, resulting from neuron overmigration and formation of an extracortical layer that resembles a bumpy cobblestone surface [10] , [11] . There are several vertebrate dystroglycanopathy models [12] ; however, a Drosophila model has not been developed. Previously, we have reported that Drosophila can serve as a great system to study muscular dystrophies and Dg deficiencies lead to muscle and nervous system disorders [13] , [14] . Drosophila Dg has distinct functions from Dys, and apart from its role in muscle maintenance it is involved in energy homeostasis, photoreceptor differentiation and neuromuscular junction establishment [14] , [15] , [16] , [17] , [18] . In addition, Dg deficiency has been shown to alter the microRNA (miRNA) profile, providing a link between the DGC and regulation of messenger RNA and protein levels [19] . Dg can be detected in various tissues in mammals and in Drosophila [13] , [20] , [21] . In both vertebrates and invertebrates, there are numerous Dg gene transcripts listed in GenBank, but it is not known why there is so much variation in the protein isoforms and what are regulatory events, including post-transcriptional control, which give rise to the mature, sugar-decorated protein. The broad expression pattern and the multiple cellular processes that Dg is being discovered to play a role in indicate that it can be considered as an ECM housekeeping gene (reviewed in ref. 3 ). Therefore, it is logical that there are various forms of regulation available to manage its levels, especially in the brain, where the exactitude of ECM–cell adhesion is particularly important for brain compartmentalization and greatly contributes to the brain complexity. Now we report that precise levels of Dg per se are critical, as lower levels slow down neuronal stem cell division, while higher levels accelerate proliferation and perturb neuron differentiation. Interestingly, altered Dg levels lead to formation of cobblestone-like structures that outgrow the normal contour of the ECM-defined brain space. This phenotype is similar to the brain cortex abnormalities associated with dystroglycanopathies in humans, implying that Drosophila Dg mutants can serve as a model for cobblestone lissencephaly. We have found that misregulation of Dg affects the distribution of major cell adhesion proteins, which presumably alters cell–ECM interaction, consequently resulting in abnormal tissue assembly. The intensity of the cobblestone-like phenotype is proportional to the amount and the duration of Dg protein misregulation. Dg is subjected to alternative 3′-UTR processing, and our evidence suggests that this is a mechanism allowing for its partial visibility to the miR-310s complex of miRNAs. This regulation is critical in response to cell shape rearrangements that take place during neuronal stem cell division, neuron differentiation, and brain morphogenesis. As a consequence of the miR-310s regulation, only a portion of Dg mRNAs with an extended 3′-UTR can be targeted, preventing Dg levels from being reduced below a certain threshold that would affect nervous system development. In addition, miR-310s levels are sensitive to those of Dg and nitric oxide (NO) signalling alike, indicating a Dg-NO- miR-310s regulatory loop. As NO signalling regulates miRNA gene expression and the cellular localization of NO signalling components per se depends on Dg, it implies that Dg is involved indirectly in transcriptional activation of its own repressors, the miR-310s . Thus, this study is an example of the proposed perceptive-executive mechanism that manages the precision of protein amounts: the information about the higher ECM receptor Dg levels is relayed via signalling that induces transcription of miRNAs. miRNAs can postranscriptionally regulate only a fraction of Dg mRNA with an alternative 3′-UTR , reducing the variance of the target and readjusting its levels via a negative feedback loop. We believe that this phenomenon might be indicative of a broader regulatory mechanism that could be in play to regulate ECM receptor levels in response to cell shape rearrangements in general. High levels of Dg result in cobblestone-like brain Multiple studies imply that Dg is not only the transmembrane component of the DGC, but also is a well-designed platform that allows communication with many interacting proteins to modulate multiple cellular processes. Thus, we postulate that Dg levels need to be tightly controlled. To test this hypothesis, we used a previously established Drosophila muscular dystrophy model, where it was shown that Dg deficit leads to age-dependent muscle defects [13] , [16] , [17] . Now we tested Dg developmental requirements and found that Dg loss retards pre-adult development ( Fig. 1a ) and affects mutant animals’ viability ( Fig. 1b ), while its overexpression with a ubiquitous Gal4 driver ( tub-Gal4 ) appears to be deadly ( Fig. 1c ). As Dg has been shown to play important roles in muscle and nervous tissues, we wanted to dissect whether this lethality was due to the requirement for exact Dg levels in muscles or in the nervous system using different tissue-specific drivers (expression exemplified in Supplementary Fig. 1 ). Increasing Dg levels in the muscle did not affect viability, but in the nervous system caused high levels of embryonic lethality ( Fig. 1c ), suggesting that there might be a need to control Dg levels, specifically in the nervous system. 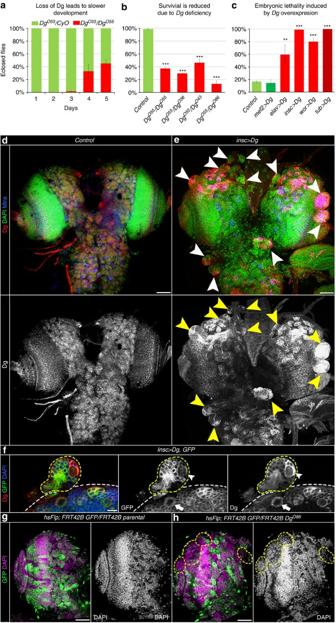Figure 1: Proper Dg levels are important forDrosophilaviability and normal brain morphology. (a) In general,Dgloss-of-function animals develop slower, as adult flies eclose 3–4 days later then their heterozygous siblings. (b) Loss of Dg leads to decreased viability, as more than one half of Dg-deficient flies die during development (embryogenesis, larval and pupal stages). The AVE±AD is reported. Two independent crosses for each allelic combination were analysed. Statistics were calculated using two-way tables and theχ2-test. (c)Dgoverexpression in the nervous system (elav>Dg,insc>Dg,wor>Dg) and ubiquitously (tub>Dg) cause high embryonic lethality. Embryos with increased muscle expression of Dg (mef>Dg) are not affected. The AVE±s.d. is reported. Three to six biological replicates were done and the two-tailed Student’st-test was used to test for statistical significance (see alsoSupplementary Table 1). (d) InControl, the larval brain has a smooth outline. (e) Overexpression of Dg using pan-neuronal driver (insc>Dg) results in the appearance of dense rounded structures that outgrow the normal shape of the brain (arrowheads). (f) Dynamic expression of the nervous system driver (insc-Gal4) results in a non-uniform pattern of lump formation. Marking the expression pattern of theinsc-Gal4driver with GFP and Dg (insc-Gal4; UAS-CD8:GFP,UAS-Dg) and co-staining with anti-GFP and anti-Dg antibodies reveals that some of the NBs have low (arrow) while others have high (arrowhead) expression levels of both GFP and Dg, and that the size of lumps appears to correlate with the strength of Dg overexpression. (g) Parental control clones (hsFlp; FRT42B GFP/FRT42B)are marked by the absence of GFP. (h) Induction of Dg loss-of-function clones (hsFlp; FRT42B GFP/FRT42B DgO86) causes abnormal clustering between clonal (Dg deficient) and non-clonal (normal levels of Dg) cells, resulting in peculiar three-dimensional brain organization. This cobblestone-like phenotype occurs with the frequency ~42% (see alsoSupplementary Table 2). White dashed lines indicate the normal boundary of the brain. Yellow dashed lines indicate brain outgrowths. *P≤0.05, **P≤0.01, ***P≤0.001. Scale bar, 25 μm (d,e,g,h) and 10 μm (f). Figure 1: Proper Dg levels are important for Drosophila viability and normal brain morphology. ( a ) In general, Dg loss-of-function animals develop slower, as adult flies eclose 3–4 days later then their heterozygous siblings. ( b ) Loss of Dg leads to decreased viability, as more than one half of Dg-deficient flies die during development (embryogenesis, larval and pupal stages). The AVE±AD is reported. Two independent crosses for each allelic combination were analysed. Statistics were calculated using two-way tables and the χ 2 -test. ( c ) Dg overexpression in the nervous system ( elav>Dg , insc>Dg , wor>Dg ) and ubiquitously ( tub>Dg ) cause high embryonic lethality. Embryos with increased muscle expression of Dg ( mef>Dg ) are not affected. The AVE±s.d. is reported. Three to six biological replicates were done and the two-tailed Student’s t -test was used to test for statistical significance (see also Supplementary Table 1 ). ( d ) In Control , the larval brain has a smooth outline. ( e ) Overexpression of Dg using pan-neuronal driver ( insc>Dg ) results in the appearance of dense rounded structures that outgrow the normal shape of the brain (arrowheads). ( f ) Dynamic expression of the nervous system driver ( insc-Gal4 ) results in a non-uniform pattern of lump formation. Marking the expression pattern of the insc-Gal4 driver with GFP and Dg ( insc-Gal4; UAS-CD8:GFP , UAS-Dg ) and co-staining with anti-GFP and anti-Dg antibodies reveals that some of the NBs have low (arrow) while others have high (arrowhead) expression levels of both GFP and Dg, and that the size of lumps appears to correlate with the strength of Dg overexpression. ( g ) Parental control clones ( hsFlp; FRT42B GFP/FRT42B) are marked by the absence of GFP. ( h ) Induction of Dg loss-of-function clones ( hsFlp; FRT42B GFP/FRT42B Dg O86 ) causes abnormal clustering between clonal (Dg deficient) and non-clonal (normal levels of Dg) cells, resulting in peculiar three-dimensional brain organization. 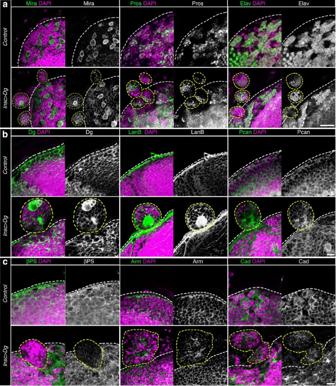Figure 2: Dg overexpression causes non-tumorous brain outgrowths resulting from abnormal interaction of neuronal cells with the ECM. (a) Cobblestone-like malformations, which result from Dg ectopic expression in nervous system, are not tumours, as each structure contains one NB marked by the neuronal stem cell-specific marker Miranda (Mira+) per cobblestone. Marking with ganglion mother cell (GMC) and neuronal markers, Prospero and Elav respectively, demonstrates typical numbers of GMCs marked with Prospero (Pros+) and differentiated neurons (Elav+), when compared withControl, indicating that asymmetry of neuronal stem cell division and major differentiation processes are not affected. (b) Overexpression of Dg influences the distribution of cell adhesion proteins: the transmembrane ECM receptor Dg, the ECM proteins LanB, Pcan; heterophilic cell adhesion protein β-integrin (β-PS), the β-Catenin homologue Armadillo (Arm) and homophilic cell adhesion protein DE-Cadherin (Cad), when compared withControl, suggesting that the above described malformed brain phenotype results from abnormal interaction of neuronal cells with the ECM. White dashed lines indicate the normal boundary of the brain. Yellow dashed lines indicate brain outgrowths. Scale bar, 20 μm (a) and 10 μm (b,c). This cobblestone-like phenotype occurs with the frequency ~42% (see also Supplementary Table 2 ). White dashed lines indicate the normal boundary of the brain. Yellow dashed lines indicate brain outgrowths. * P ≤0.05, ** P ≤0.01, *** P ≤0.001. Scale bar, 25 μm ( d , e , g , h ) and 10 μm ( f ). Full size image Next, we wanted to understand what is the cause for the lethality. Dg overexpression in the nervous system resulted in a peculiar phenotype: dense cellular masses that overgrow the normal brain contour ( Fig. 1d,e ; arrowheads). The majority of Dg-overexpressing mutants die during larval stages; however, a few escapers make it to adulthood. Their brains also contained lumps ( Supplementary Fig. 2a–c ), but in a lesser quantity than observed on average in larval brains, suggesting that the penetrance of the brain overgrowth phenotype is variable. We also noted that lump-like structures found within one brain could be irregular in size ( Fig. 1e ). As neuronal Gal4 drivers may have somewhat variable expression patterns, the size of the overgrowths should correlate with the localized strength of driver expression. To test this, we co-expressed green fluorescent protein (GFP) as a marker for the efficiency of Gal4 expression and full-length Dg (insc-Gal4>UAS GFP, UAS Dg). We observed that clusters with the highest GFP levels (the strongest Gal4 activity, the highest Dg expression) produced qualitatively larger lumps ( Fig. 1f ), substantiating a direct correlation between the Dg amount and brain malformation. Similar effects were observed on Dg overexpression by pan-neuronal (elav-Gal4) and neuronal stem-cell-specific (wor-Gal4) drivers: some of the neuronal stem cells (neuroblasts (NBs)) expressed high, while others moderate levels of Dg ( Supplementary Fig. 2d–f ). Interestingly, NBs and their progeny that had similar amounts of Dg protein clustered together and grouped into separate lumps, indicating that lump size and assembly correlate with Dg levels. To specify the time course of the abnormal lump formation and provide evidence that this effect is cell-autonomous, we took advantage of the temporally inducible FRT–FLP system to obtain Dg overexpression clonal cells. Early Dg-overexpressing clones (analysed 1 day after clone induction) did not show any obvious abnormalities; however, after 3 days, clonal cells that overexpressed Dg started to aggregate and formed clearly outlined three-dimensional masses, beginning to separate from the rest of the brain tissue ( Supplementary Fig. 2g,h ). Notably, induced Dg-deficient cellular clones or Dg downregulation ( tub>DgRNAi ) also resulted in similar brain malformations; however, the observed phenotype was milder in comparison with its overexpression ( Fig. 1h and Supplementary Table 2 ). Thus, regardless of whether Dg levels are increased or decreased, the cobblestone-like brain phenotype appears. These data demonstrate the following: (1) the precision of Dg expression levels affects brain morphology; (2) the severity of the observed brain defect depends on the amount and duration of abnormal Dg levels; and (3) the effect of Dg misregulation on the brain lump formation is cell autonomous, which together implies that Dg levels must be stabilized for normal brain development. Dg non-tumorous outgrowths caused by cell adhesion defects Next, we wanted to understand the nature of these brain defects. First, we suspected that the observed Dg-linked brain lumps were tumours that occurred due to neuronal stem cell division and/or neuron differentiation defects. However, staining of mutant brains with the antibody against the neuronal stem cell and neuron-specific markers proved that asymmetry of neuronal stem cell division and the major differentiation processes are not affected ( Fig. 2a ). Thus, we concluded that these lumps were not tumours. Figure 2: Dg overexpression causes non-tumorous brain outgrowths resulting from abnormal interaction of neuronal cells with the ECM. ( a ) Cobblestone-like malformations, which result from Dg ectopic expression in nervous system, are not tumours, as each structure contains one NB marked by the neuronal stem cell-specific marker Miranda (Mira + ) per cobblestone. Marking with ganglion mother cell (GMC) and neuronal markers, Prospero and Elav respectively, demonstrates typical numbers of GMCs marked with Prospero (Pros + ) and differentiated neurons (Elav + ), when compared with Control , indicating that asymmetry of neuronal stem cell division and major differentiation processes are not affected. ( b ) Overexpression of Dg influences the distribution of cell adhesion proteins: the transmembrane ECM receptor Dg, the ECM proteins LanB, Pcan; heterophilic cell adhesion protein β-integrin (β-PS), the β-Catenin homologue Armadillo (Arm) and homophilic cell adhesion protein DE-Cadherin (Cad), when compared with Control , suggesting that the above described malformed brain phenotype results from abnormal interaction of neuronal cells with the ECM. White dashed lines indicate the normal boundary of the brain. Yellow dashed lines indicate brain outgrowths. Scale bar, 20 μm ( a ) and 10 μm ( b , c ). Full size image Second, we hypothesized that Dg’s interaction with the ECM could be responsible for the cobblestone-like brain phenotype and the strength of the ECM–cell interaction could contribute to abnormal lump formation. Similar to that in vertebrates, Drosophila Dg contains two functional domains: the extracellular domain that connects to the ECM and the cytoplasmic domain that interacts with Dys and other DGC proteins [13] . To establish which functional part of Dg is responsible for the observed brain overgrowth phenotype, we overexpressed a truncated Dg version that lacks the extracellular domain ( DgΔExD , Supplementary Fig. 3a ). Importantly, misregulation of this version of Dg had no effect on the brain shape ( Supplementary Fig. 3a–c ), suggesting that the altered brain morphology due to abnormal Dg levels results from impaired Dg-ECM communication. Therefore, we analysed the expression pattern of cell adhesion proteins in tandem with Dg overexpression. In contrast to neuronal cell differentiation markers, we found the distribution of major cell adhesion receptors and ECM molecules to be highly abnormal. According to the genotype, Dg levels were extremely upregulated in the brain outgrowths ( Fig. 2b ). In vertebrates, Dg is a key receptor for the major class of ECM proteins, laminins, and defects in α-Dg posttranslational modifications cause aberrant interactions with different laminins, causing muscular dystrophy development and exacerbation [22] , [23] , [24] , [25] . As it has not been shown that in Drosophila brain Dg interacts with laminins, we performed co-immunoprecipitation analysis with the brain-specific GFP-tagged Dg ( Supplementary Fig. 3d,e ) and the ECM protein LamininB (LanB), demonstrating that Dg can act as a laminin receptor in the fly brain ( Supplementary Fig. 3e ). Moreover, LanB was notably upregulated in the forming cysts ( Fig. 2b ). Another ECM protein, Perlecan (Pcan) that binds Dg in vitro [26] was also upregulated and differentially localized ( Fig. 2b ). LanB and Pcan are major macromolecular components of the neural lamella, the extracellular net-like ECM sheet that outlines the developing brain. On Dg misregulation, lumps protrude above this ECM-formed outermost brain layer ( Fig. 2b ). At the same time, levels of the major extracellular receptor required for cell–ECM interaction, integrin (βPS), is drastically reduced in these structures compared with Control ( Fig. 2c ). It is known that Dg competes with integrins for ECM binding, and levels of both Dg and integrins are co-dependently readjusted at the transcriptional level via the ECM [27] . Thus, Dg misregulation alters the βPS integrin expression pattern and ECM composition, such as LanB and Pcan levels and distribution. In addition, higher Dg levels cause reduction as well as mislocalization of cell–cell adhesion proteins at the cellular membrane (β-catenin=Arm and E-cadherin=Cad, Fig. 2c ). Together, these data demonstrate that the Dg-malformed brain phenotype is associated with abnormal cell–ECM and cell–cell adhesion. Thus, on Dg misregulation, neuronal cells express altered levels of ECM molecules and cell adhesion receptors, which cause abnormal interaction of these cells with the rest of the brain tissue. As a result of selective cell adhesion, these cells with aberrant Dg levels cluster together, forming lumps that are dissociated from other cells and are pushed out from the brain. Notably, similar cobblestone brain structure is a characteristic of lissencephaly type II in humans suffering from dystroglycanopathies [10] , [28] , which are also caused by abnormal α-Dg interaction with the ECM. Resemblance of the brain phenotypes proposes that Drosophila Dg mutants can be used as a model to study these neurodevelopmental diseases. Dg can be accessible to miRNA regulation via a variable 3′-UTR Owing to the evidence that Dg needs to be precisely regulated in the nervous system, we next studied the mechanism of how Dg can be regulated there. The Dg transcript has the possibility of having at least two different 3′-UTRs according to FlyBase annotation ( Fig. 3a ). Recently, it has been shown that 3′-UTRs of metazoan mRNAs contain various regulatory motifs that influence mRNA stability, localization and translational efficiency, affecting numerous cellular processes [29] , [30] . It is logical to hypothesize that longer 3′-UTRs may contain regulatory motifs that can be used to fine-tune spatiotemporal signalling. When we probed Dg complementary DNA with primers that recognize a region belonging to both the short and long 3′-UTR and a region of only the long 3′-UTR , we found that ~60% of Dg transcripts have the longer 3′-UTR version ( Fig. 3b ). mRNA in situ hybridization using a probe with primers that recognize the long 3′-UTR showed expression in the brain, imaginal disks, muscles and other tissues ( Fig. 3c and Supplementary Fig. 4a ) and no obvious difference in expression patterns was observed between the Dg protein [13] , [14] , [16] and the Dg long 3′-UTR mRNA. 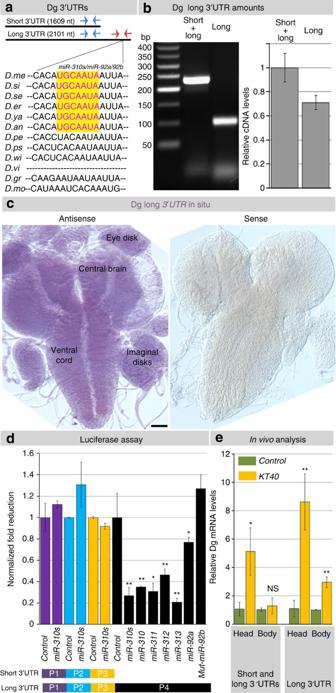Figure 3:Dg’s variable3′-UTRallows for alternative targeting bymiR-310s. (a) Schematic drawing of the variable Dg3′-UTRs, the short and the long that is extended by an additional 491 bp. Arrows mark the location of primers used to detectDgmRNA with both the shorter and the long3′-UTR, and just the long3′-UTR. (b) PCR analysis of cDNA from whole flies with primers that recognize the region of the long3′-UTR, and the region common for both long and short3′-UTRversions ofDgtranscript show that ~60% of theDgmRNA has the longer3′-UTRregion present (analysis was done taking into the account primer efficiencies). (c)In situhybridization against the long3′-UTRregion shows that the long3′-UTRcontainingDgmRNA is present in the larval brain. Scale bar, 25 μm. (d) Consistent with the fact that only the extended version of theDg 3′-UTRhas themiR-310sbinding site, no reduction in luciferase activity is observed when fragments of theDg 3′-UTRcommon for the short and longDg 3′-UTRs(but without the miR-310s binding site) were assayed (P1, P2 and P3). When the reporter gene fused to an appropriate fragment of theDglong3′-UTRcontaining themiR-310sputative binding site is assayed (P4), a decrease in luciferase activity is observed even in the absence of miRNA transgenes (~1.5-fold), presumably due to endogenous levels of targeting miRNAs in the cells. When also transformed with plasmids expressingmiR-310s(all), individual cluster miRNAs andmiR-92a(but notmut-miR-92bthat contains a single point mutation in the seed sequence, CACTGCA instead of CATTGCA), a further decrease in luciferase activity (~1.3- to 4.7-fold) is seen (Supplementary Table 3). (e)KT40mutants (loss ofmiR-310s) have elevated levels of totalDgmRNA detected by primers that recognize both short and long3′-UTRs. This upregulation is more pronounced when primers specifically against the long3′-UTRregion or RNA extracts from heads were used (Supplementary Table 4). Three to five independent biological experiments were analysed. The AVE±s.d. is reported and two-tailed Student’st-test was used to test for statistical analyses: *P≤0.05, **P≤0.01, ***P≤0.001, NS, not significant. Figure 3: Dg ’s variable 3′-UTR allows for alternative targeting by miR-310s . ( a ) Schematic drawing of the variable Dg 3′-UTR s, the short and the long that is extended by an additional 491 bp. Arrows mark the location of primers used to detect Dg mRNA with both the shorter and the long 3′-UTR , and just the long 3′-UTR . ( b ) PCR analysis of cDNA from whole flies with primers that recognize the region of the long 3′-UTR , and the region common for both long and short 3′-UTR versions of Dg transcript show that ~60% of the Dg mRNA has the longer 3′-UTR region present (analysis was done taking into the account primer efficiencies). ( c ) In situ hybridization against the long 3′-UTR region shows that the long 3′-UTR containing Dg mRNA is present in the larval brain. Scale bar, 25 μm. ( d ) Consistent with the fact that only the extended version of the Dg 3′-UTR has the miR-310s binding site, no reduction in luciferase activity is observed when fragments of the Dg 3′-UTR common for the short and long Dg 3′-UTRs (but without the miR-310s binding site) were assayed (P1, P2 and P3). When the reporter gene fused to an appropriate fragment of the Dg long 3′-UTR containing the miR-310s putative binding site is assayed (P4), a decrease in luciferase activity is observed even in the absence of miRNA transgenes (~1.5-fold), presumably due to endogenous levels of targeting miRNAs in the cells. When also transformed with plasmids expressing miR-310s (all), individual cluster miRNAs and miR-92a (but not mut-miR-92b that contains a single point mutation in the seed sequence, CACTGCA instead of CATTGCA), a further decrease in luciferase activity (~1.3- to 4.7-fold) is seen ( Supplementary Table 3 ). 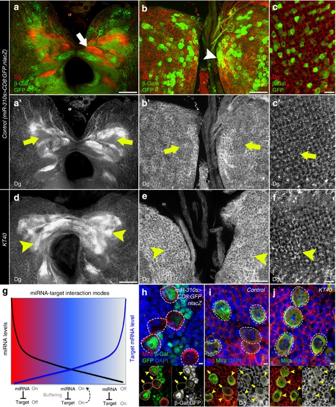Figure 4: Complementary and non-complementary expression ofDgandmiR-310s. (a–c) Analysis of the expression patterns of Dg protein and themiR-310srevealed that there are two possible modes of howmiR-310scan regulate Dg levels. Axonal bundles in the central brain neuropils express Dg andmiR-310sin a mutually exclusive pattern (a), meaning that there is no regulation or that a miRNA completely downregulates its target. Cells located at the brain surface express both, themiR-310sand Dg (b), meaning that a miRNA buffers its target levels. A similar co-expression pattern is observed in the visual system (c). As a readout ofmiR-310sexpression, we used a Gal4 insertion in themiR-310slocus,P(GawB)NP4255(referred to asmiR-310s-Gal4) from Kyoto DGRC.miR-310sexpression was visualized by anti-β-Gal and anti-GFP antibodies in the brain expressing nuclear lacZ and membrane GFP under control of themiR-310spromoter (miR-310s-Gal4/+; UAS-mCD8-GFP, UAS-nLacZ/+). Dg was visualized by antibody staining. (d–f). To test how themiR-310sregulate Dg in the brain, we analysed Dg expression inKT40mutants. InmiR-310smutants, the Dg expression pattern is altered in the central brain region (d), more axonal bundles expressed Dg in the absence ofmiR-310s, confirming the idea thatmiR-310sand Dg are expressed in the ‘off/on’ mode in the central brain axons. Similarly, Dg expression levels are increased in the brain surface neuronal and photoreceptor cells (e,f) in comparison withControl(a’,b’andc’), suggesting that themiR-310salso buffer Dg levels. (g) Scheme representing the architecture of the miRNA-target network: expression tuning and expression buffering (modified from ref.33). (h) Neuronal cells express themiR-310sin a selective manner (arrows and arrowheads). (i,j) Dg is expressed in all of the cells of the larval brain with somewhat variable levels (arrows and arrowheads). Dg expression levels are increased in all neuronal cells in the larval brain ofmiR-310smutant (j, arrowheads). White dashed lines outline NBs inh–j. Scale bar, 25 μm (a,b,d,e), 5 μm (c,f), 2 μm (h–j). ( e ) KT40 mutants (loss of miR-310s ) have elevated levels of total Dg mRNA detected by primers that recognize both short and long 3′-UTR s. This upregulation is more pronounced when primers specifically against the long 3′-UTR region or RNA extracts from heads were used ( Supplementary Table 4 ). Three to five independent biological experiments were analysed. The AVE±s.d. is reported and two-tailed Student’s t -test was used to test for statistical analyses: * P ≤0.05, ** P ≤0.01, *** P ≤0.001, NS, not significant. Full size image As Dg has an alternative 3′-UTR , it can be reasoned that there is a regulatory function for this diversity. Theoretically, by varying the 3′-UTR length, Dg becomes more or less visible to regulation by miRNAs. For example, the short 3′-UTR does not have, while the Dg-extended 3′-UTR has, a predicted binding site for a family of miRNAs, the miR-310s ( miR-310, miR-311, miR-312, miR-313 ), miR-92a and miR-92b , which we found to be Dg-dependent in our miRNA microarray screen [19] . The long 3′-UTR is evolutionarily conserved and present among all Drosophila species, but the conservation in the sequence corresponding to the seed of the newly evolved miR-310s miRNA family ( Fig. 3a ) developed along with the emergence of the miR-310s , via miR-92a/b duplication, around 53 million years ago [31] . As the conservation of the corresponding sequence necessary for targeting by the miR-310s appeared at the same time as these miRNAs emerged, we thought that it might be physiologically relevant and, next, we examined whether the miR-310s can target Dg. First, to determine whether the miR-310s target Dg’s extended 3′-UTR , we assayed a luciferase reporter gene with different 3′-UTR fragments in Drosophila S2R+ cells ( Supplementary Table 3 ). The luciferase assay showed that the miR-310s can target Dg via the extended 3′-UTR in vitro and confirmed the miR-310 seed sequence specificity ( Fig. 3d ). Next, we also verified that Dg could be targeted by the miR-310s in Drosophila tissue, where we analysed ovarian follicle cell clones that ectopically express the miR-310s ( Supplementary Fig. 4c ). Together, these data demonstrate that the miR-310s can downregulate Dg in vitro and in vivo via its long 3′-UTR . Finally, we tested whether miR-310s -based regulation of Dg has a functional role in living animals. We found that miR-310s loss-of-function mutants, KT40 (ref. 32 ) have higher levels of total Dg mRNA detected by primers that recognize the short and long 3′-UTRs and only the long 3′-UTR ( Fig. 3e ). This dramatic increase in Dg expression could be also seen at the protein level measured by western blot analysis ( Supplementary Fig. 4b ). Dg mRNA levels were increased even more in heads alone, indicating that Dg regulation is primarily occurring in the head. Moreover, Dg mRNA levels with the long 3′-UTR in the head increased ~8.5 times, presumably due to Dg targeting in the central brain and eyes ( Fig. 3e ). The determining mechanism for transcribed 3′-UTR length is ambiguous, but in the presence of mixed 3′-UTRs certain levels of Dg would be maintained via invisibility to miR-310s targeting, offering protection from Dg deficit. We next sought to define whether Dg and the miR-310s have similar expression in the nervous system and whether they share other phenotypes. miR-310s and Dg expression in the nervous system is dynamic We analysed the expression pattern of Dg and the miR-310s. Interestingly, we found that there are two possible modes of how miR-310s can regulate Dg levels: axonal bundles in the central brain neuropils express Dg and miR-310s in a mutually exclusive pattern ( Fig. 4a–a′ ), while cells located at the brain surface or in the developing visual system express both the miRNA and its target Dg ( Fig. 4b–c′ ). miRNA functions can be classified into two categories: expression tuning (when a miRNA is setting the mean of the expression level of the target gene resulting in the ‘on-off’ expression pattern) and expression buffering (when a miRNA reduces the variance of the target where the miRNA and its target are co-expressed). These two functions are independent and can co-exist ( Fig. 4g , reviewed in ref. 33 ). Dg protein expression analysis in miR-310s deficient flies shows that miR-310s and Dg could interact in the expression tuning and buffering modes ( Fig. 4d–f ). Figure 4: Complementary and non-complementary expression of Dg and miR-310s . ( a – c ) Analysis of the expression patterns of Dg protein and the miR-310s revealed that there are two possible modes of how miR-310s can regulate Dg levels. Axonal bundles in the central brain neuropils express Dg and miR-310s in a mutually exclusive pattern ( a ), meaning that there is no regulation or that a miRNA completely downregulates its target. Cells located at the brain surface express both, the miR-310s and Dg ( b ), meaning that a miRNA buffers its target levels. A similar co-expression pattern is observed in the visual system ( c ). As a readout of miR-310s expression, we used a Gal4 insertion in the miR-310s locus, P(GawB)NP4255 (referred to as miR-310s-Gal4 ) from Kyoto DGRC. miR-310s expression was visualized by anti-β-Gal and anti-GFP antibodies in the brain expressing nuclear lacZ and membrane GFP under control of the miR-310s promoter ( miR-310s-Gal4/+; UAS-mCD8-GFP, UAS-nLacZ /+). Dg was visualized by antibody staining. ( d – f ). To test how the miR-310s regulate Dg in the brain, we analysed Dg expression in KT40 mutants. In miR-310s mutants, the Dg expression pattern is altered in the central brain region ( d ), more axonal bundles expressed Dg in the absence of miR-310s , confirming the idea that miR-310s and Dg are expressed in the ‘off/on’ mode in the central brain axons. Similarly, Dg expression levels are increased in the brain surface neuronal and photoreceptor cells ( e , f ) in comparison with Control ( a’ , b’ and c’ ), suggesting that the miR-310s also buffer Dg levels. ( g ) Scheme representing the architecture of the miRNA-target network: expression tuning and expression buffering (modified from ref. 33 ). ( h ) Neuronal cells express the miR-310s in a selective manner (arrows and arrowheads). ( i , j ) Dg is expressed in all of the cells of the larval brain with somewhat variable levels (arrows and arrowheads). Dg expression levels are increased in all neuronal cells in the larval brain of miR-310s mutant ( j , arrowheads). White dashed lines outline NBs in h – j . Scale bar, 25 μm ( a , b , d , e ), 5 μm ( c , f ), 2 μm ( h – j ). Full size image Dg, detected by antibody staining, is broadly expressed in the nervous system and, as expected, its levels are variable. For example, some neuronal stem cells had higher, while others had lower or undetectable, Dg amounts ( Fig. 4i ). The fluctuating Dg levels were also characteristic for other cells in the brain, suggesting that its levels vary, possibly during different stages of the neuronal lifecycle, such as cell division or neuron maturation. We analysed in detail neuronal cells that co-express Dg and the miR-310s . If Dg levels fluctuate, they must be re-adjusted; therefore, we analysed in more detail neuronal cells that co-express Dg and the miR-310s . miR-310s expression (marked by nuclear lacZ, miR-310s>nlacZ , driven by the endogenous miR-310s promoter) was detected in a subset of each Dg-expressing cell type on the brain surface and their expression levels were also fluctuating ( Fig. 4h and Supplementary Fig. 5a ). However, on miR-310s loss, Dg levels were visibly increased in all brain cells ( Fig. 4i,j ). Comparison of the expression patterns shows that Dg and the miR-310s are expressed in some of the same cell types and their levels are dynamic, confirming the expression-buffering mode of miR-310s -Dg interaction ( Fig. 4g ). Considering that Dg levels are critical for proper formation of the nervous tissue and that the miR-310s can regulate only isoforms of the Dg mRNA with the extended 3′-UTR (~60% of total Dg mRNA), we propose that the miR-310s buffer the expression of its target Dg against fluctuation, perhaps dynamically. Dg and miR-310s fine-tune the mitotic index of neuronal stem cells As miRNA-based regulation could offer additional safeguarding, we next investigated the biological significance of Dg buffering by these miRNAs in the nervous system. We tested whether similar phenotypes are associated with Dg deregulation and the miR-310s loss in the developing brain. Importantly, we found that the miR-310s loss-of-function mutant, similar to Dg loss- and gain-of- function mutants, exhibits cobblestone brain ( Supplementary Table 2 ), suggesting that Dg buffering by the miR-310s via Dg’s extended 3′-UTR is relevant for brain development. Dg misregulation affects the amounts of multiple proteins involved in cell adhesion ( Fig. 2c ), intensity of which modifies multiple aspects of the cellular lifecycle, including cell proliferation [6] , [34] . In particular, we found that the loss of Dg results in a decreased number of mitotically active neuronal stem cells, NBs ( Fig. 5a–d ). Moreover, Dg overexpression in miR-310s -expressing cells and miR-310s deficiency caused a significant overproliferation rate, while Dg deficit substantially decreased the NB mitotic index ( Fig. 5d ). These data show that managing the levels of miR-310s and the ECM receptor Dg is important to fine-tune the mitotic index of neuronal stem cells. We hypothesize that this is because NB cell divisions are normally accompanied by cell–ECM and cell–cell contact rearrangements requiring a proper ECM composition that depends on Dg amounts. 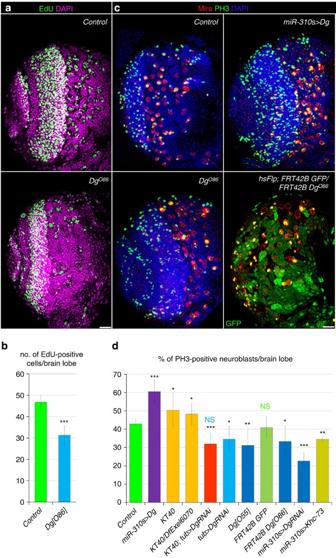Figure 5: ThemiR-310sand Dg regulate proliferation of neuronal stem cells. (a,b) On Dg deficiency, the frequency of actively dividing cells (S phase, marked by EdU) is significantly decreased in the larval brain in comparison withControl.Fourteen to 16 lobes were counted per genotype. (c,d) On Dg deficiency (DgO86, DgO55andFRT42B DgO86clones) or Dg downregulation using RNAi driven by the ubiquitous and the dynamicmiR-310s Gal4drivers (tub>DgRNAiandmiR-310s>DgRNAi), the frequencies of NBs in M phase (marked by PH3 and Mira, yellow) are significantly decreased.Dgoverexpression inmiR-310s-expressing cells results in overproliferation defects comparable to the defects occurring due to the loss of themiR-310s(KT40andKT40/DfExel6070), the mitotic index of larval brain NBs significantly increased compared withControl.Six to 17 lobes were counted per genotype. To prove that this decrease in the number of PH3- and EdU-positive NBs is not due to increased apoptosis induced by the absence of the principal ECM receptor, activated Caspase3 staining was performed inDgloss-of-function (DgO55) mutants and no elevated numbers of apoptotic cells per brain were observed; four out of nine brains had one apoptotic cell where the maximum number of positive cells seen was four in one brain, which was similar toControl. Dg knockdown cannot rescue themiR-310sdeletion phenotype (compareKT40; tub>DgRNAiandtub>DgRNAi), plausibly because RNAi-based downregulation of Dg is more efficient than Dg upregulation resulting frommiR-310sloss. Overexpression of another confirmedmiR-310starget,Khc-73(ref.32) (miR-310s-Gal4/UAS-Khc-73), decreases the mitotic index, which is opposite to the increase seen inKT40andmiR-310s-Gal4/UAS-Dgmutants. These data confirm previous findings about the role for Khc-73 in NB division; however, this shows that the increased proliferation phenotype observed inmiR-310sloss-of-function mutants is not due to anmiR-310s-Khc-73interaction in NBs. See alsoSupplementary Table 5. The AVE±s.d. are reported and significance was tested using the two-tailed Student’st-test: *P≤0.05, **P≤0.01, ***P≤0.001, NS, not significant. Scale bar, 25 μm. Figure 5: The miR-310s and Dg regulate proliferation of neuronal stem cells. ( a , b ) On Dg deficiency, the frequency of actively dividing cells (S phase, marked by EdU) is significantly decreased in the larval brain in comparison with Control. Fourteen to 16 lobes were counted per genotype. ( c , d ) On Dg deficiency ( Dg O86 , Dg O55 and FRT42B Dg O86 clones) or Dg downregulation using RNAi driven by the ubiquitous and the dynamic miR-310s Gal4 drivers ( tub>DgRNAi and miR-310s>DgRNAi ), the frequencies of NBs in M phase (marked by PH3 and Mira, yellow) are significantly decreased. Dg overexpression in miR-310s -expressing cells results in overproliferation defects comparable to the defects occurring due to the loss of the miR-310s ( KT40 and KT40/DfExel6070 ), the mitotic index of larval brain NBs significantly increased compared with Control. Six to 17 lobes were counted per genotype. To prove that this decrease in the number of PH3- and EdU-positive NBs is not due to increased apoptosis induced by the absence of the principal ECM receptor, activated Caspase3 staining was performed in Dg loss-of-function ( Dg O55 ) mutants and no elevated numbers of apoptotic cells per brain were observed; four out of nine brains had one apoptotic cell where the maximum number of positive cells seen was four in one brain, which was similar to Control . Dg knockdown cannot rescue the miR-310s deletion phenotype (compare KT40; tub>DgRNAi and tub>DgRNAi ), plausibly because RNAi-based downregulation of Dg is more efficient than Dg upregulation resulting from miR-310s loss. Overexpression of another confirmed miR-310s target, Khc-73 (ref. 32 ) ( miR-310s-Gal4/UAS-Khc-73 ), decreases the mitotic index, which is opposite to the increase seen in KT40 and miR-310s-Gal4/UAS-Dg mutants. These data confirm previous findings about the role for Khc-73 in NB division; however, this shows that the increased proliferation phenotype observed in miR-310s loss-of-function mutants is not due to an miR-310s-Khc-73 interaction in NBs. See also Supplementary Table 5 . The AVE±s.d. are reported and significance was tested using the two-tailed Student’s t -test: * P ≤0.05, ** P ≤0.01, *** P ≤0.001, NS, not significant. Scale bar, 25 μm. Full size image miR-310s regulation of Dg is necessary in the visual system Other processes, accuracy of which highly depends on ECM composition, are neuron differentiation and axon pathfinding. Therefore, next we analysed whether the miRNA-based regulation of Dg levels takes place in the visual system, where Dg previously has been shown to play an essential role in terminal differentiation of Drosophila photoreceptor neurons [13] , [16] . We found that only some of the photoreceptor neurons within ommatidium express the miR-310s and that Dg levels are miR-310s dependent; in miR-310s mutants, Dg was accumulated and its cellular localization was affected in these cells ( Fig. 6a–c and Supplementary Fig. 5 ). 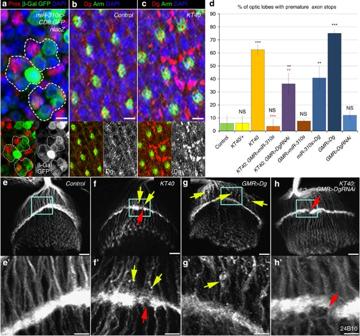Figure 6: Dg regulation by themiR-310sis important for proper photoreceptor axon guidance during development of the visual system. (a) TheDrosophilacompound eye consists of ~800 ommatidia that each contains 8 photoreceptor neurons or R-cells (R1–8). ThemiR-310sare expressed variably in photoreceptor neurons visualized with anti-β-Gal and anti-GFP (miR-310s-Gal4/+; UAS-mCD8-GFP, UAS-nLacZ/+), and the R7 marker Prospero (Pros)57(white dashed lines outline a single ommatidium). Note that nuclear β-Gal and membrane GFP do not always co-localize: β-Gal and GFP have different protein turnover rates, suggesting dynamicmiR-310sexpression. (b) Dg is expressed in all photoreceptor neurons. (c) Dg levels aremiR-310sdependent; inKT40photoreceptor cells, Dg is accumulated and its cellular localization is affected. However, due to the nature of the used reporter that visualizesmiR-310sexpression via lacZ and GFP proteins, which depends on the time of their production and degradation, it is not feasible to evaluate the correspondingmiR-310sand Dg protein levels in a given cell. See alsoSupplementary Fig. 5b. (d) The bar graph represents percentages of defective axon projections in the indicated genotypes. The experiment was conducted using three different bouts of progeny from independent crosses (biological replicate). Each experimental round consisted of between 5 and 20 optic lobe examinations being marked as disturbed or normal to generate an experimental percentage per biological replicate. The AVE±s.d. is reported and the two-tailed Student’st-test was used to test for statistical significance: *P≤0.05, **P≤0.01, ***P≤0.001, NS, not significant. Black stars—compared withControl (w1118), red stars—compared withKT40mutants. SeeSupplementary Table 6. (e,f) In contrast toControl(d), in theKT40mutants (e) axon terminations in the lamina plexus have gaps and breaks (red arrows), reminiscent of the photoreceptor axon pathfinding defects inDgloss-of-function mutants, but additionally mutants have premature axon stops (yellow arrows). (g) Ectopic expression ofDgusingmiR-310s-Gal4andGMR-Gal4drivers recapitulates the premature axon stops noted inKT40mutants only. (h) The premature termination phenotype and lamina plexus gaps can be rescued inKT40mutants by overexpressing themiR-310s(KT40; GMR>miR-310s;Supplementary Table 6). Accordingly, premature axon termination can be rescued by reduction of Dg (KT40; GMR>DgRNAi) in the eye.e’–h’are enlarged regions outlined in cyan ine–h.Scale bar, 2 μm (a–c), 10 μm (e–h) and 5 μm (e’–h’). Figure 6: Dg regulation by the miR-310s is important for proper photoreceptor axon guidance during development of the visual system. ( a ) The Drosophila compound eye consists of ~800 ommatidia that each contains 8 photoreceptor neurons or R-cells (R1–8). The miR-310s are expressed variably in photoreceptor neurons visualized with anti-β-Gal and anti-GFP ( miR-310s-Gal4/+; UAS-mCD8-GFP, UAS-nLacZ/+ ), and the R7 marker Prospero (Pros) [57] (white dashed lines outline a single ommatidium). Note that nuclear β-Gal and membrane GFP do not always co-localize: β-Gal and GFP have different protein turnover rates, suggesting dynamic miR-310s expression. ( b ) Dg is expressed in all photoreceptor neurons. ( c ) Dg levels are miR-310s dependent; in KT40 photoreceptor cells, Dg is accumulated and its cellular localization is affected. However, due to the nature of the used reporter that visualizes miR-310s expression via lacZ and GFP proteins, which depends on the time of their production and degradation, it is not feasible to evaluate the corresponding miR-310s and Dg protein levels in a given cell. See also Supplementary Fig. 5b . ( d ) The bar graph represents percentages of defective axon projections in the indicated genotypes. The experiment was conducted using three different bouts of progeny from independent crosses (biological replicate). Each experimental round consisted of between 5 and 20 optic lobe examinations being marked as disturbed or normal to generate an experimental percentage per biological replicate. The AVE±s.d. is reported and the two-tailed Student’s t -test was used to test for statistical significance: * P ≤0.05, ** P ≤0.01, *** P ≤0.001, NS, not significant. Black stars—compared with Control (w 1118 ), red stars—compared with KT40 mutants. See Supplementary Table 6 . ( e , f ) In contrast to Control ( d ), in the KT40 mutants ( e ) axon terminations in the lamina plexus have gaps and breaks (red arrows), reminiscent of the photoreceptor axon pathfinding defects in Dg loss-of-function mutants, but additionally mutants have premature axon stops (yellow arrows). ( g ) Ectopic expression of Dg using miR-310s-Gal4 and GMR-Gal4 drivers recapitulates the premature axon stops noted in KT40 mutants only. ( h ) The premature termination phenotype and lamina plexus gaps can be rescued in KT40 mutants by overexpressing the miR-310s ( KT40; GMR>miR-310s ; Supplementary Table 6 ). Accordingly, premature axon termination can be rescued by reduction of Dg ( KT40; GMR>DgRNAi ) in the eye. e’ – h’ are enlarged regions outlined in cyan in e – h. Scale bar, 2 μm ( a – c ), 10 μm ( e – h ) and 5 μm ( e’ – h’ ). Full size image Photoreceptor neurons undergo complex reorganization during development: migration, axon growth and projection, and synapse formation, and all of these events are associated with dynamic cell shape rearrangements that are highly dependent on cell adhesion (reviewed in ref. 1 ). Ectopic Dg expression in photoreceptor neurons and specifically in miR-310s -expressing cells recapitulates the premature axon stops noted in miR-310s mutants ( Fig. 6d–h ). Importantly, reduction of Dg specifically in photoreceptor cells and miR-310s overexpression can rescue the premature axon termination phenotype in the miR-310s mutant background ( Fig. 6h ), showing that regulation of exact Dg levels via the miR-310s is important for proper photoreceptor neuron differentiation. In summary, these data show that in the nervous system maintaining precise levels of the ECM receptor, Dg, is particularly important, as Dg abnormal levels affect distribution of cell adhesion proteins, subsequently influencing neuronal stem cell division speed, neuron differentiation and nervous tissue morphology. Dg regulates miR-310s expression via a negative feedback loop If the miR-310s are assigned to buffer Dg only when required, it is possible that miRNA expression itself could be sensitive to higher levels of the target. Thus, we hypothesize that the miR-310s promoter can be responsive to Dg amounts, which would reassure homeostatic Dg levels. To confer the responsiveness of miR-310s expression to abnormal Dg levels, we overexpressed Dg with the dynamic miR-310s promoter that is shared by all miRNAs in the miR-310s family and measured the levels of a representative miRNA, miR-312 . We observed an ~5-fold increase in miR-312 levels due to Dg overexpression, reciprocally, Dg loss results in lower levels of miR-312 ( Fig. 7a ). This effect can also be visualized on the cellular level; for example, when in Control , the majority of ommatidia in the eye imaginal disk contain two cells that have the transcriptionally active miR-310s promoter, and Dg overexpression results in more cells actively expressing the miR-310s ( Fig. 7b,c ). These data imply that the miR-310s and Dg are in a negative feedback loop, where expression of miRNAs is induced in response to higher levels of their target ( Fig. 7d ). 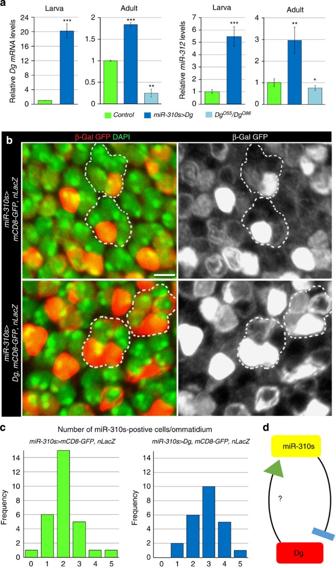Figure 7:miR-310sexpression depends on Dg levels. (a)DgmRNA levels are upregulated in flies where Dg is expressed under control of themiR-310sendogenous promoter. High levels of Dg coincide with increased, while lack of Dg with decreased amounts ofmiR-312, one of the miRNAs from themiR-310scomplex. Three independent biological replicates were analysed. The AVE±s.d. is reported and the two-tailed Student’st-test was used to test for statistical significance: *P≤0.05, **P≤0.01, ***P≤0.001. SeeSupplementary Table 4. (b)Dgoverexpression (miR-310s-Gal4/+; UAS-Dg/UAS-mCD8-GFP, UAS-nLacZ) inmiR-310s-expressing cells marked by anti-GFP and β-Gal staining leads to an increased number of cells positive for GFP and β-Gal in comparison with animals that do not overexpressDg(miR-310s-Gal4/+; UAS-mCD8-GFP, UAS-nLacZ). Scale bar, 2 μm. (c) Histogram showing the frequency ofmiR-310s-positive cells/ommatidium (miR-310s-Gal4/+; UAS-mCD8-GFP, UAS-LacZ, n=29 ommatidia,miR-310s-Gal4/+; UAS-Dg/UAS-mCD8-GFP, UAS-nLacZ, n=24). The two-tailed Mann–WhitneyU-test predicts statistical significance withP=0.0027. (d) Schematic model showing themiR-310sand Dg regulation in a negative feedback loop. Figure 7: miR-310s expression depends on Dg levels. ( a ) Dg mRNA levels are upregulated in flies where Dg is expressed under control of the miR-310s endogenous promoter. High levels of Dg coincide with increased, while lack of Dg with decreased amounts of miR-312 , one of the miRNAs from the miR-310s complex. Three independent biological replicates were analysed. The AVE±s.d. is reported and the two-tailed Student’s t -test was used to test for statistical significance: * P ≤0.05, ** P ≤0.01, *** P ≤0.001. See Supplementary Table 4 . ( b ) Dg overexpression ( miR-310s-Gal4/+; UAS-Dg/UAS-mCD8-GFP, UAS-nLacZ ) in miR-310s -expressing cells marked by anti-GFP and β-Gal staining leads to an increased number of cells positive for GFP and β-Gal in comparison with animals that do not overexpress Dg ( miR-310s-Gal4/+; UAS-mCD8-GFP, UAS-nLacZ ). Scale bar, 2 μm. ( c ) Histogram showing the frequency of miR-310s -positive cells/ommatidium ( miR-310s-Gal4/+; UAS-mCD8-GFP, UAS-LacZ, n =29 ommatidia, miR-310s-Gal4/+; UAS-Dg/UAS-mCD8-GFP, UAS-nLacZ, n =24). The two-tailed Mann–Whitney U -test predicts statistical significance with P =0.0027. ( d ) Schematic model showing the miR-310s and Dg regulation in a negative feedback loop. Full size image Dg regulates miR-310s expression via NO signalling Dg is a transmembrane receptor and the question of how it can regulate miR-310s expression at the transcriptional level needs to be answered. Previously, it has been shown in vertebrates that the DGC acts as a scaffold responsible for the membrane localization of signalling proteins ( Fig. 8a ). In particular, Dg, via Dys or Dystrobrevin, anchors Syntrophins (Syn) that bind neuronal NO synthase and, as a result, regulate generation of NO [35] , [36] . NO nitrosylates the histone deacetylases that regulate gene transcription and in vertebrate muscles the Dys-Syn-neuronal NO synthase signalling pathway regulates histone modifications that control transcription of miRNA genes [37] . Recently, we showed that in Drosophila , Dg-Dys-Syn signalling also controls the miRNA expression profile [19] . Therefore, we decided to test whether Dg-mediated regulation of miR-310s expression occurs via NO signalling. 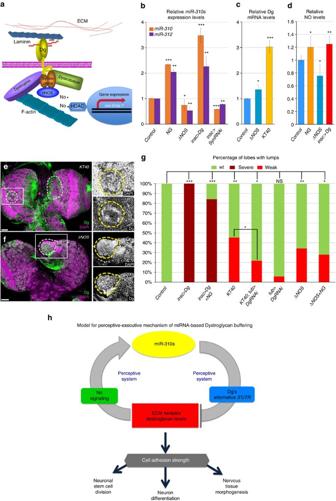Figure 8:miR-310sgene expression depends on Dg and NO signalling to adjust Dg via a feedback loop. (a) Schematic drawing represents the DGC and its potential role in regulatingmiR-310sthrough NO signalling. (b)miR-310andmiR-312levels are increased on treatment of wild-type larvae with the NO donor, NG and are decreased inΔNOSandinsc>SynRNAimutants. (c)DgmRNA levels are increased inΔNOSandKT40larvae (Supplementary Table 4). (d) NG treatment, similar to Dg overexpression (insc>Dg), leads to significantly higher NO levels, while inΔNOSmutants relative NO levels are significantly decreased. SeeSupplementary Table 7. (e,f) Similar to Dg overexpression, brains with lumps that have high levels of Dg can be observed inKT40(d) andΔNOS(e) mutants. Note that the observed cobblestone phenotype is milder than in Dg-overexpressing flies. Scale bar, 25 μm. (g) Bar graph represents percentages of brain lobes that contain lumps in the indicated genotypes. The observed mutant phenotype can be rescued inKT40mutants by downregulation of Dg with ubiquitous driver (KT40; tub>DgRNAi). SeeSupplementary Table 2. (h) Schematic model showing that dynamic expression ofmiR-310sin the nervous system can be regulated by Dg and NO signalling via a negative feedback loop. Three to six biological replicates (b–d) and 16–108 brain lobes from 3 to 5 independent biological experiments (g) were analysed. The AVE±s.d. is reported. To calculate the statistical significance the two-tailed Student’st-test was used inbandc, two samplez-test indand two-way tables and theχ2-test ing: *P≤0.05, **P≤0.01, ***P≤0.001. Figure 8: miR-310s gene expression depends on Dg and NO signalling to adjust Dg via a feedback loop. ( a ) Schematic drawing represents the DGC and its potential role in regulating miR-310s through NO signalling. ( b ) miR-310 and miR-312 levels are increased on treatment of wild-type larvae with the NO donor, NG and are decreased in ΔNOS and insc>SynRNAi mutants. ( c ) Dg mRNA levels are increased in ΔNOS and KT40 larvae ( Supplementary Table 4 ). ( d ) NG treatment, similar to Dg overexpression ( insc>Dg ), leads to significantly higher NO levels, while in ΔNOS mutants relative NO levels are significantly decreased. See Supplementary Table 7 . ( e , f ) Similar to Dg overexpression, brains with lumps that have high levels of Dg can be observed in KT40 ( d ) and ΔNOS ( e ) mutants. Note that the observed cobblestone phenotype is milder than in Dg-overexpressing flies. Scale bar, 25 μm. ( g ) Bar graph represents percentages of brain lobes that contain lumps in the indicated genotypes. The observed mutant phenotype can be rescued in KT40 mutants by downregulation of Dg with ubiquitous driver ( KT40; tub>DgRNAi ). See Supplementary Table 2 . ( h ) Schematic model showing that dynamic expression of miR-310s in the nervous system can be regulated by Dg and NO signalling via a negative feedback loop. Three to six biological replicates ( b – d ) and 16–108 brain lobes from 3 to 5 independent biological experiments ( g ) were analysed. The AVE±s.d. is reported. To calculate the statistical significance the two-tailed Student’s t -test was used in b and c , two sample z -test in d and two-way tables and the χ 2 -test in g : * P ≤0.05, ** P ≤0.01, *** P ≤0.001. Full size image First, we addressed whether the outgrowth phenotype induced by Dg overexpression depends on the DGC being a platform for NO signalling. To test this, we analysed Dys expression in the mutant brains and found that on Dg overexpression Dys amounts at the protein (but not mRNA) levels are significantly increased ( Supplementary Fig. 6 ). Plausibly, Dys is stabilized when bound to Dg and it is anchored to the membrane. The increase of both major components of the complex, specifically in brain lumps, allows the assumption that the outgrowth phenotype induced by overexpression of Dg does occur through the DGC. Next, we tested whether the levels of miR-310s expression depend on DGC-NO signalling. To provide the mechanistic evidence for NO regulation of miR-310s -Dg expression, we fed Drosophila nitroglycerin (NG) as a NO donor and measured the levels of miR-310 and miR-312 . Importantly, NG treatment significantly increased, while NO synthase deficiency [38] (ΔNOS) or Syn downregulation in the nervous system (insc>SynRNAi) significantly decreased these miRNAs levels, conferring the miR-310s promoter responsiveness to NO signalling ( Fig. 8b ). Even more, similar to miR-310s mutants, Dg levels were upregulated on NO synthase deficiency ( Fig. 8c ). As Dg is an anchor protein required for localization of NO signalling components, its amounts potentially can regulate NO signalling strength and play an indirect role in control of at least miR-310s expression. Therefore, we tested NO levels in flies that overexpress Dg in the nervous system and observed that relative NO levels were increased, which was comparable to the amounts measured on NG treatment, while in NOS-deficient flies these were significantly reduced ( Fig. 8d ). In addition, miR-310s and NOS deficiencies phenotypically copied, to a lesser extent, the cobblestone brain phenotype caused by Dg overexpression ( Fig. 8e,f ). Consistently, the milder brain phenotype in KT40 and ΔNOS mutants, relative to nervous system overexpression of Dg (insc>Dg) , correlated with the measured Dg protein amounts ( Supplementary Fig. 4b ), again correlating that the severity of the brain dysplasia directly depends on the extent of Dg deregulation. Similar to Dg mutant brains, cobblestone-like structures observed on miR-310s deficiency were also associated with aberrant cell adhesion protein expression ( Supplementary Fig. 7 ). Importantly, the miR-310s mutant brain phenotype could be significantly rescued by reducing Dg levels ( Fig. 8g ). In addition, NO treatment had some positive effect on the brain outgrowth phenotype in Dg-overexpressing and NOS -deficient flies ( Fig. 8g ); however, it could not fully rescue it. This implies that some early NO-dependent developmental processes are irreversible and could not be repaired by transient NG administration. Taken together, these data show that the miR-310s promoter is responsive to the presence of higher amounts of Dg and NO signalling. This proposes that Dg is involved in transcriptional activation of the miR-310s via NO signalling, while NO signalling and the miR-310s in turn attenuate Dg abundance via a negative feedback loop. In summary, our data propose a novel perceptive-executive model for protein levels adjustment: it is perceptive, because it senses high levels of a critical protein, and it is executive, because it results in transcriptional activation of miRNAs that target the protein to restore its normal levels ( Fig. 8h ). As we showed, this regulation is potentially of great importance for stabilization of Dg expression levels, which modulates multiple cellular processes in the developing nervous system ( Fig. 8h ). As a consequence of miR-310s regulation, only a portion of Dg mRNAs with an extended 3′-UTR can be targeted, preventing Dg levels from being reduced below a certain threshold, which also is damaging for brain formation. Potentially, having a form of the target that is insensitive to miRNAs (alternatively processed 3′-UTR ) allows adjustment of the target amount only to a critical level. Thus, the variability of 3′-UTR sequences has great significance in regulation of gene expression, where miRNAs act as managers of this extra layer of precision. Currently, the mechanisms coordinating alternative 3′-UTR processing for specific mRNA isoforms remain elusive; therefore, it would be important to understand what signalling controls the specifics of Dg 3′-UTR processing. Intriguingly, we found that the majority of the non-integrin ECM receptors have alternative 3′-UTRs that can be subjected to differential miRNA targeting ( Table 1 ). This implies that the presented perceptive-executive model might be a more general buffering mechanism to readjust levels of essential molecules. Further, more detailed molecular evidence is required for the proposed here mechanism of protein expression regulation. Table 1 3′-UTRs of known Drosophila ECM receptors. Full size table Alternative 3′-UTRs are common, sometimes tissue-specific, and often correlate with developmental stages, becoming shorter as the animal ages [30] . Recent bioinformatic work has shown that a high number of vertebrate mRNAs are alternatively polyadenylated and cleaved, leading to transcripts with different 3′-UTR lengths [39] . Interestingly, the longest 3′-UTRs among adult tissues are found in the brain [40] , [41] , [42] and 3′-UTR length also correlates with cell proliferation: tumour cells contain shorter 3′-UTRs [43] . Moreover, proliferating cells can have conserved mRNA transcripts with shorter 3′-UTRs in diverse cell types and tissues, and interestingly expression of the full-length 3′-UTRs results in reduced protein levels that can be reversed by mutating predicted miRNA target sites [44] . Therefore, the variability of 3′-UTR sequences offers an additional step, safeguarding the precision of gene expression where miRNAs play a key role. In this study, we report that Dg is subject to variable 3′-UTR processing and such processing determines its visibility to at least one family of miRNAs—the miR-310s . Interestingly, the 3′-UTR of the human Dg ( DAG1) gene contains multiple miRNA binding sites and most of them are evolutionary conserved between vertebrates, suggesting that miRNA-based regulation of this important housekeeping gene might also take place in vertebrate organisms. Prior studies in vertebrate muscle demonstrated that a signalling pathway involving DGC-regulated histone modification manages the proper transcription of miRNA genes [37] . In addition, regulation of mRNA levels is changed in human muscular dystrophies, correlating with mis-expressed miRNA–mRNA modules [45] . Interestingly, restoring of NO signalling or using histone deacetylase inhibitors return mis-expressed miRNAs to normal levels in mdx mice [46] and affectively ameliorate muscular dystrophy [47] . This proposes that the DGC via regulation of NO signalling maintains equilibrium between acetylation and deacetylation of histones and has an impact on muscle maintenance and/or the regenerative potential of muscle stem cells. In a miRNA microarray screen conducted on dystrophic flies, we found that on DGC deficit the expression profile of multiple miRNAs is altered [19] . Moreover, some of these miRNAs are predicted to be involved in multiple processes in the nervous system [19] . In addition, our study is the first report showing that Dg at least in Drosophila can be regulated posttranscriptionally via miRNAs in the nervous system. Here we propose that in the nervous system, Dg is able to regulate miRNA gene expression presumably via a NO-dependent mechanism. This implies that Dg and NO signalling can actively adjust epigenetic characteristics of neuronal cells. As Dg is also a signal-transducing module involved in crosstalk between the internal and external environments, this study suggests that Dg is involved in highly managed regulation of gene expression required to adapt cellular homeostasis that is compromised under dystrophic conditions. It would be important in the future to study in more detail how Dg via NO signalling manages gene expression in the nervous system. We propose that Drosophila can be used as a model organism to study cobblestone lissencephaly, because Dg misregulation mutants present all typical syndromes associated with dystroglycanopathy: muscle degeneration [13] , [14] , cobblestone brain and eye defects. Dystroglycanopathies are very pleiotropic, their associated pathologies range from very severe to few or no structural defects [48] , [49] . This wide symptomatic range can be explained by the nature of the mutations causing these neuromuscular disorders, which occur in multiple proteins that decorate the Dg glycoprotein with different sugars in a tissue-specific manner; other Dg modifications, such as phosphorylation and proteolysis, also have a profound effect on its physiological functions [6] , [23] . Thus, the common mechanism underlying the assortment of the defects observed in secondary dystroglycanopathies is abnormal cellular interaction with the ECM, composition of which is also altered due to abnormal α-Dg posttranslational modifications. Dg interacts with various laminins in a tissue- and cell type-specific manner, and abnormal α-Dg posttranslational modifications generally alter the strength of neuron adhesion to the ECM. As our findings show that either decreased or increased Dg levels result in the cobblestone brain, we propose that proper brain architecture formation requires the intensity of Dg-coordinated cell–ECM interactions to be accurate. As cells produce their own ECM, there is bidirectional signalling between the extra- and intracellular machinery. For example, we showed that in Drosophila , Dg modulates the levels of the ECM protein laminin non-cell and cell autonomously, thus adjusting the ECM constitution to be in accordance with the amounts of Dg expressed by the cell [27] . The precision of cell adhesion protein expression is extremely important in the nervous system. Brain development, compartmentalization and even synapse formation rely on the quantity and quality of cell adhesion molecules expressed by different types of neurons [50] . Based on expression patterns, we propose that there are different requirements for Dg as a cell adhesion receptor during different stages of neuron differentiation: first, to properly cluster, axons of fully differentiated neurons express certain levels of cell adhesion molecules; therefore, they have low, high or no Dg; second, to properly divide and differentiate, NBs, ganglion mother cells and not yet fully differentiated neurons readjust Dg levels according to their life cycle. In addition, we found that Dg is an important neuronal stem cell cycle regulator, as its misregulation leads to loss of cell cycle control in the brain. Together, our data show that the accuracy of neuronal proliferation, differentiation and axon pathfinding greatly depend on Dg levels and that miRNAs are candidates to buffer the levels of Dg expression against fluctuation in these processes. Overall, we believe that our Drosophila cobblestone lissencephaly model will allow for the better understanding of the molecular basis of dystroglycanopathies. Fly strains and genetics Fly stocks were maintained at 25 °C on a standard cornmeal-agar diet unless otherwise stated. The following Drosophila fly stocks were used: wild-type strain Oregon-R-C and w 1118 that were used as Controls ; GMR-Gal4 , elav-Gal4 , tub-Gal4 , act-Gal4 , D42-Gal4 , 24B-Gal4 , MHC-Gal4 , wor-Gal4 , insc-Gal4 , the deficiency spanning the miR-310s locus DfExel6070 (Bloomington Drosophila Stock Center); and UAS-Khc-73 DP00530 (ref. 51 ). We used a Gal4 insertion in the miR-310s locus, P(GawB)NP4255 (referred to as miR-310s-Gal4 ), from Kyoto DGRC to analyse the miR-310s complex expression pattern [32] . We observed no phenotypes in homozygous flies with this insert and measured the levels of miR-312 to be the same as in Oregon R flies. The miR-310s overexpression line ( UAS-miR-310s/TM6 ) and deletion of miR-310s cluster line, KT40 (ref. 32 ). For overexpression of Dg, we used transgenic lines containing the following constructs: UASt-Dg , which includes Dg full-length coding sequence, followed by truncated Dg 3′-UTR (670 bp, does not contain the miR-310s binding site); UASt-DgΔExD , which encodes truncated Dg that lacks the ECM binding domain [52] ; and UASt-Dg:GFP , which contains GFP-tagged full-length Dg (used for immunoprecipitation analyses) [15] . For loss-of-function experiments, we used Dg mutants, Dg O86 /CyO , Dg O43 /CyO , Dg O38 /CyO and Dg O55 /CyO , and NOS mutant, Nos Δ15 (referred to as ΔNOS ) [38] . The UAS-mCD8-GFP, UAS -nLacZ flies were kindly provided by Frank Hirth, and hsFlp; Stau-GFP; act<FRT-CD2-FRT<Gal4, UAS-GFP by Wu-Min Deng. To analyse the specificity of the phenotypes and to eliminate the possibility of a second site mutation, heteroallelic flies were analysed. All mutants and transgenes used in the experiments were compared with the control of the similar genetic background. Lethality and development speed analyses For embryonic lethality, flies were placed on agar plates with apple juice and allowed to lay eggs at 25 °C for 3–5 h and then the total number of eggs was counted. Embryos on plates were allowed to develop, and after 48 h the number of eggs that did not hatch was counted. The lethality was calculated by dividing the number of eggs that did not hatch by the total number of eggs. To analyse the viability and developmental delay caused by Dg loss-of-function Dg O86 /CyO , Dg O43 /CyO and Dg O38 /CyO lines were crossed to Dg O55 /CyO and the numbers of Dg homozygous versus Dg over CyO balancer heterozygous flies were counted during 5 days after flies started to eclose. CyO/+ flies were intercrossed and their progeny were scored as Controls. As Cy is a lethal mutation, the expected ratio of Cy versus non- Cy flies should be 2:1. The percentage of survival was calculated as ratio between the number of eclosed homozygous flies divided by half of the number of eclosed flies with the Cy wing phenotype and multiplied by 100%. Immunohistochemistry Tissues were dissected and fixed in 4% formaldehyde. Antibody staining was performed as described before [14] . The following antibodies were used: rabbit anti-Dg C-term [52] (1:2,000), rabbit anti-Dg ex8 (ref. 53 ) (1:500), mouse anti-22C10, anti-β-Gal, anti-Elav, anti-βPS Integrin, anti-Pcan, anti-Arm, anti-Pros and rat anti-DE-Cad (1:50; Developmental Studies Hybridoma Bank), chicken anti-GFP (1:2,000; Abcam), rabbit anti-β-Gal (1:1,000; Invitrogen), rabbit anti-Phospho-Histone 3 (anti-PH3, 1:2,000; Upstate Biotechnologies), guinea pig anti-Miranda (gift from Andreas Wodarz, 1:1,000), rabbit anti-Caspase3 (1:200; Abcam), rabbit anti-LanB (1:1,000, Abcam ab47651), rabbit anti-Dys186 (gift from Lee Fradkin), Alexa 488/568 goat anti-mouse, Alexa 488/568/633 goat anti-rabbit, Alexa 488 goat anti-mouse, Alexa 568 goat anti-guinea pig, Alexa 488 goat anti-chicken (1:500; Invitrogen). Samples were mounted on slides in 70% glycerol, 2% n-propyl gallate, 1 × PBS and analysed using a confocal microscope (Zeiss LSM 700). Quantification of staining intensities was done using the Zeiss software. Histology To prepare Drosophila tissue sections, flies were immobilized in collars in the required orientation and fixed in Carnoy fixative solution (6:3:1, ethanol: chloroform:acetic acid) at 4 °C overnight. Tissue dehydration and embedding in paraffin was performed as described previously [54] . Ten-micrometre histological sections were prepared using a Hyrax M25 (Zeiss) microtome and stained with haematoxylin and eosin. All chemicals for these procedures were obtained from Sigma Aldrich. Analysis was done using a light microscope (Zeiss). Induction of loss- and gain-of-function clones Females of genotype hsFlp; act<FRT-CD2-FRT<Gal4, UAS-GFP were crossed to males of genotype UAS-miR-310s/TM6 . Two- to three-day-old females of the correct genotype were subjected to 1 h 37 °C heat-shock treatment for 2 consecutive days and put to fresh food with wet yeast for 3 days at which point ovaries were dissected and subjected to immunohistochemistry. To obtain Dg gain-of-function clones, hsFlp; act<FRT-CD2-FRT<Gal4, UAS-GFP were crossed either to OregonR (Control) or UAS-Dg flies and to obtain Dg loss-of-function clones; females of genotype hsFlp; FRT42B Ubi-GFP/CyO were crossed to males of genotype w 1118 ; FRT42B Dg O86 /CyO or to parental FRT 42B as a control. F1 larvae from the cross were heat shocked for 2 h at 37 °C for 2 consecutive days and dissected as L3 to analyse the brains. EdU labelling To label cells that are in S phase, brains from L3 larvae where dissected in Schneider’s Drosophila Medium (Life Technologies) and incubated in medium containing 0.01 μM EdU (5-ethyl-2′-deoxyuridine) for 1 h followed by fixation in 4% formaldehyde in 1 × PBS for 20 min. Next, brain sections were washed two times with PBT (0.2% Triton X in 1 × PBS) (20 min each) and blocked with PBTB (1 × PBT, 0.2% bovine serum albumin, 5% normal goat serum, 0.05% sodium azide) for 30 min. Labelling of EdU-positive cells was performed using Click-iT EdU Alexa Fluor 555 Imaging Kit (Invitrogen/Molecular Probes) according to the manufacturer’s protocol, followed by standard antibody staining protocol. Nitroglycerin feeding Thirsty 3- to 7-day-old adult flies were put overnight in vials containing filter paper soaked in 5% sucrose with 0.2 ng μl −1 NG (VWR EHERLA15586000AL) or just 5% sucrose ( Control ). 0.2 ng μl −1 was the concentration of NG on which the lethality was <5%. Larvae were kept in vials with standard fly food supplemented with 500 μl of 5% sucrose with or without 0.2 ng μl −1 NG. L3 larvae were collected ~12 h after NG treatment. Measurement of NO levels To measure NO levels OxiSelect in Vitro Nitric Oxide Assay Kit was used (Cell Bioloabs STA-802). Measurements of total nitrite/nitrate amounts were done according to the manufacturer’s protocol. Samples were prepared from three whole larvae in the standard western blotting lysis buffer. In situ hybridization Probes were designed to target the longer region of the 3′-UTR annotated in Flybase release FB2012_02 to belong to the Dg-RD transcript. Primers used to generate an ~350 bp sense fragment were: forward—5′- TAATACGACTCACTATAGGG TCACGCAGTTAGTTATTCTC-3′ and reverse—5′-CACATAGACAAGAGTAAGTACAG-3′, where the underlined region corresponds with the T7 RNA polymerase promoter region. Primers used to generate an ~350 bp anti-sense fragment were: forward—5′-TCACGCAGTTAGTTATTCTC-3′ and reverse—5′- TAATACGACTCACTATAGGG CACATAGACAAGAGTAAGTACAG-3′. Genomic DNA was PCR amplified using the above primers. One microgram of DNA in a 20-μl reaction was converted into RNA using a DIG RNA labelling kit (2 μl 10 × transcription buffer, 2 μl 10 × NTP labelling mixture (Roche), 1 μl RNase inhibitor (Applied Biosystems) and 2 μl of T7 RNA polymerase (New England Biolabs)). The reaction was carried out for 2 h at 37 °C. The solution was then treated with 2 μl of DNase1 (Invitrogen) for 15 min at 37 °C, and the reaction was stopped by the addition of 2 μl of 0.2 M EDTA. One microlitre of the solution was run on an agarose gel to ensure that the RNA product was of the expected size. The probes were then stored at −20 °C in 10 μl of 1 M Tris pH 7.5 and 100 μl of hybridization buffer (50% formamide, 25% 20 × SSC, 5 mg ml −1 Torula yeast RNA (Sigma), 0.1% Tween 20) until their use. Tissues were dissected, fixed for 30 min in 4% formaldehyde in PBS, dehydrated and stored at −20 °C overnight or longer. Tissues were then rehydrated, treated for 30 min to 1 h with Proteinase K solution (50 μg ml −1 Proteinase K in 50 mM Tris-HCl pH 7.5, 50 mM EDTA), and post-fixed in 4% formaldehyde in PBT for 30 min. Tissues were prehybridized for 1 h in hybridization buffer. Hybridization was carried out overnight at 60 °C with 2 μl per 100 μl of probe in hybridization buffer. Post hybridization washing was done at 62 °C with 3 subsequent 20-min washes with hybridization solution, 50/50 v/v hybridization solution/PBT, PBT. Tissues were then blocked for 1 h in Western Block (Sigma). Anti-DIG was diluted 1:2,000 in block and incubated with tissues overnight at 4 °C. Colorimetric detection was done with 10 μl ml −1 NBT (Roche) in staining buffer (0.05 M Tris pH 9.5, 0.05 M MgCl 2 , 0.1 M NaCl, 0.1% Tween 20) for ~30–45 min. Analysis was done using Zeiss LSM 700 microscope. PCR amplification of cDNAs cDNA was generated as described above and subjected to standard PCR on a T100 Thermocycler (Bio-Rad) using the appropriate primers as described above to target the short and long Dg 3′-UTR , and to target the long Dg 3′-UTR . The PCR products were separated via electrophoresis on a 2% agarose gel. Densitometric analysis was used to determine the relative amounts of PCR products. Amplification efficiency was determined via densitometric analysis of the relative levels of unused primers for each reaction visualized at the bottom of the gel. PCR product levels were adjusted for the respective primer efficiencies and compared against one another to determine relative levels. The PCR product generated from primers that target both the short and long 3′-UTR were used as the normalizing quantity. Reverse-transcription quantitative PCR Total RNA was extracted using Trizol reagent (Invitrogen) following the manufacturer’s protocol and treated with DNase1 (Invitrogen). To detect miRNA levels TaqMan microRNA assays (Applied Biosystems) were used to reverse transcribe from RNA and amplify cDNA specific to miR-310 , miR-311 , miR-312 , miR-313 , miR-92a , miR-92b and 2S rRNA as an endogenous control on a StepOne Plus thermocycler (Applied Biosystems). Quantitative PCR (qPCR) was done using the Taqman qPCR master mix (Applied Biosystems). For the determination of transcript levels, mRNA was converted into cDNA using the High-Capacity reverse transcription kit (Applied Biosystems) following the manufacturer’s directions. cDNA for Dg mRNA was amplified using the SYBR green master mix (Applied Biosystems). To detect Dg cDNA corresponding to the 3′-UTR long isoform, the forward and reverse primers were used respectively: 5′-TGGCTTCAATTGAGCGAGCT-3′ and 5′-TCACGCAGTTAGTTATTCTC-3′ ( Fig. 3a ). To detect Dg cDNA corresponding to the 3′-UTR long and short isoforms, following forward and reverse primers were used respectively: 5′-TTCACAAGCTCCCCTTTG GA-3′ and 5′-TCATTTCCCATCCTTCATGCAAC-3′ ( Fig. 3a ). As an endogenous control for all qPCR reactions, a product was also amplified corresponding to Ribosomal Protein L32 (RpL32) with the following forward and reverse primers respectively: 5′-AAGATGACCATCCGCCCAGC-3′ and 5′-GTCGATACCCTTGGGCTTGC-3′. All reactions were run at least in triplicate with appropriate blank controls. The threshold cycle ( C T ) is defined as the fractional cycle number at which the fluorescence passes a fixed threshold. The Δ C T value is determined by subtracting the average RpL32 or 2S rRNA C T value from the average tested C T value. The ΔΔ C T value is calculated by subtracting the Δ C T of the control sample from the Δ C T of the suspect sample. The relative amount of mRNA or microRNA is then determined using the expression 2 −ΔΔCT . Luciferase reporter assay Drosophila S2R+ cells (DGRC Indiana) were seeded in a 96-well cell culture plate 1 day after splitting 1:5. Cells were transfected using the Effectene transfection reagent (Qiagen) with the following amounts: 50 ng of empty psiCHECK-2 (Promega) or 50 ng of psiCHECK-2 with the Dg-long- 3′-UTR sensor cloned in, 25 ng of act-Gal4 and/or 50 ng of the pUAST-miR test plasmid. Approximately 72 h after transfection, the cells were subjected to the Dual-Glo luciferase assay (Promega). Both firefly (control reporter) and Renilla luciferase (altered 3′-UTR experimental reporter) levels were measured to achieve optimal and consistent results. Plates were analysed on a Wallac 1,420 luminometer. Non-transfected cells were used for blank subtraction from raw luminescence counts. The experimental reporter ( Renilla luciferase) counts were divided by control reporter counts ( Firefly luciferase) to determine the ratio of experimental/control reporter luminescence. The ratio of Renilla luciferase activity in the presence of the psiCHECK-2-Dg-3′-UTR plasmid with an appropriate Dg 3′-UTR fragment (P1–P4) was divided by the fold decrease in the presence of the empty psiCHECK-2 plasmid without the presence of transfected pUAST-miR plasmids to determine the downregulation ratio (control). Next, the Renilla luciferase activity was determined in the same way with the empty psiCHECK-2 and the psiCHECK-2-Dg-3′-UTR plasmid in the presence of the test pUAST-miR and the downregulation ratio between these values was calculated. The downregulation ratio of luminescence between the psiCHECK-2 plasmid and the psiCHECK-2-Dg-3′-UTR plasmid in the presence of the test pUAST-miR was then normalized to the downregulation ratio between the psiCHECK-2 plasmid and the psiCHECK-2-Dg-3′-UTR plasmid without the test pUAST-miR to determine the relative reduction in Renilla luciferase expression caused by the presence of the test miRNA. The two-tailed Student’s t -test was used to examine the significance of the effects statistically. All transfections were done three independent times to determine an average and s.e.m. The DNA plasmids pUAST-miR-310s , pUAST-miR-312 , pUAST-miR-313 , pUAST-miR-92a and pUAST-miR-92b were generated in the Lai lab [55] and obtained from the Drosophila Genomics Resource Center. To generate sensors for Dg 3′-UTR regions, fragments of interest were amplified from genomic Drosophila melanogaster DNA by PCR with primers that included enzymatic digestion sites for NotI and XhoI as follows: P1:Dg-3′-UTR : Fwd—5′- TACGTGCGGCCGC TTCGCAAATATTGGC-3′, Rev—5′- CCACCATGGCTCGAG TCCCTGAATCGAACT-3′; P2:Dg-3′-UTR: Fwd—5′- TACGTGCGGCCGC GTAGGTAGTAGTGTAGTAAG-3′, Rev—5′- CCACCATGGCTCGAG CATCAAAGGATCAGG-3′; P3:Dg-3′-UTR: Fwd—5′- TACGTGCGGCCGC TGGGACGATGGACATGTGTGC-3′, Rev—5′- CCACCATGGCTCGAG GCAGCAGGAAAGCAGCAAACC-3′; P4:Dg-long-3′-UTR : Fwd—5′- TACGTGCGGCCGC TCACGCAGTTAGTTATTCTC-3′, Rev—5′- CCACCATGGCTCGAG CACATAGACAAGAGTAAGTACAG-3′, where the additional bases for enzyme cut sites are underlined. Fragments were subsequently cloned into NotI and XhoI restriction sites downstream of the Renilla luciferase gene in the psiCHECK-2 vector (Promega). Western blotting Sample preparation and SDS–PAGE have been described previously [56] . Bio-Rad ready-made 4–20% polyacrylamide gels were used for protein separation. Proteins were transferred to polyvinylidene difluoride membranes (BioRad) using a semi-dry transfer apparatus (Bio-Rad). Primary affinity-purified anti-Dg antibodies were used at 1:30,000. Goat anti-rabbit horseradish peroxidase-conjugated antibodies (Bio-Rad) were used as detection reagents at 1:10,000. Proteins were visualized via enhanced chemiluminescence (Millipore). Densitometry analysis was performed with the ImageJ programme. Uncropped scans of western blottings are provided in Supplementary Fig. 8 . Protein extraction and immunoprecipitation Samples for immunoprecipitation were prepared from Drosophila larval brains that were homogenized and lysed in lysis buffer containing 50 mM Tris-HCl, 125 mM NaCl, 5% glycerol, 0.5% NP40, 0.25% Na-deoxycholate, 1.5 mM MgCl2, 1 mM dithiothreitol, 25 mM NaF, 1 mM Na 3 VO 4 , 1 mM EDTA, 2 mM EGTA and protease inhibitors. Samples where then centrifuged at 15,000 g for 15 min at 4 °C. Protein extracts were pre-cleared with mouse IgG-agarose beads (Sigma) at 4 °C for 1 h. Supernatants were immunoprecipitated with GFP-Trap beads (ChromoTek) following the manufacturer’s instructions. Ten per cent of total protein extracts used for immunoprecipitation was loaded as input. The presence of immunocomplexes was analysed via western blotting with LanB antibodies (1:10,000 Abcam). How to cite this article : Yatsenko, A. S. et al. miRNA-based buffering of the cobblestone-lissencephaly-associated extracellular matrix receptor dystroglycan via its alternative 3′-UTR . Nat. Commun. 5:4906 doi: 10.1038/ncomms5906 (2014).